Advances and challenges in retinoid delivery systems in regenerative and therapeutic medicine Retinoids regulate a wide spectrum of cellular functions from the embryo throughout adulthood, including cell differentiation, metabolic regulation, and inflammation. These traits make retinoids very attractive molecules for medical purposes. In light of some of the physicochemical limitations of retinoids, the development of drug delivery systems offers several advantages for clinical translation of retinoid-based therapies, including improved solubilization, prolonged circulation, reduced toxicity, sustained release, and improved efficacy. In this Review, we discuss advances in preclinical and clinical tests regarding retinoid formulations, specifically the ones based in natural retinoids, evaluated in the context of regenerative medicine, brain, cancer, skin, and immune diseases. Advantages and limitations of retinoid formulations, as well as prospects to push the field forward, will be presented. Retinoic acid (RA) signaling is one of the most important biological pathways in nature, triggered by RA interaction with nuclear receptors that control gene expression. The chemical structure of retinol (vitamin A, a RA precursor) was first described by Paul Karrer in 1931 [1] , who was awarded a Nobel Prize in 1937 for the discovery. The use of RA for skin disorders [2] and cancer treatment (acute myeloid leukemia (AML) [3] and cervical neoplasia [4] , [5] ) started in the 1960s and 1980s (Fig. 1 ). By the 2000s, RA had been incorporated in many tissue engineering scaffolds as a stem cell differentiation agent [6] , [7] . Over the last 10 years, many discoveries related to the biological role of RA in controlling the biology of hematopoietic stem cells [8] , [9] , tumor-initiating cells [10] , [11] , [12] , immune cells [13] , intestinal mucosa wound repair [14] , cancer resistance [15] , and cell reprogramming and differentiation [16] , [17] , have further stimulated the interest in this drug for many other biomedical applications. 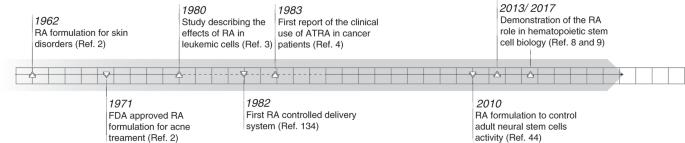Fig. 1: Milestones in RA formulations research. ATRA all-transretinoic acid, FDA Food and Drug Administration, RA retinoic acid. This interest is confirmed by more than 50 active clinical trials (according to ClinicalTrials.gov ) evaluating the effect of RA in cancer (28 trials), mostly in hematological (16 trials) and brain tumors (8 trials), skin pathologies (e.g., acne, photoaging, eczema) (5 trials), and in other conditions such as inflammation, olfactory loss, and neuropsychiatric diseases (Table 1 ). Fig. 1: Milestones in RA formulations research. ATRA all- trans retinoic acid, FDA Food and Drug Administration, RA retinoic acid. Full size image Table 1 RA formulations tested in past and ongoing clinical trials. Full size table Clinical applications of RA have highlighted three main limitations of its pharmacological use. First, RA is poorly soluble in aqueous solutions [18] and photosensitive [19] , which makes its administration challenging. Secondly, RA induces irritation when applied onto the skin and increases its catabolism, when it is administered intravenously, reducing its therapeutic efficacy [20] . Lastly, RA is involved in many biological processes and thus the systemic delivery of RA causes side effects. All these limitations motivated researchers to synthesize novel and better tolerated synthetic retinoid compounds and to develop retinoid delivery formulations based on gels, liposomes, microparticles, nanoparticles, and micro-/nanofibers, which in some cases have been modified to target-specific tissues and cells of interest [21] . Recent developments in the use of retinoid for cancer treatment [22] , [23] and differentiation studies using stem/progenitor cells [8] , [24] , as well as the development of more advanced formulations to control retinoid bioactivity [25] , [26] , make this review timely. In addition, except for a limited number of reviews, with a restricted scientific scope in retinoid formulations (treatment of skin disorders) [27] or highlighting the importance of retinoids in development (early organogenesis) [28] or for specific therapeutic applications (cancer and metabolic disease) [29] , no study has fully covered the application of retinoid formulations for diverse therapeutic and regenerative medicine applications. In this review, the role of retinoid formulations in the context of the brain, skin, immune system, and cancer applications will be discussed. For each application, the pathological context will be briefly presented as well as the effect of retinoid that was administered without any controlled release system. The reasons behind the development of retinoid formulations in each application will be presented, along with their benefits and limitations, considering retinoid solubility, photostability, biocompatibility, release profile, tissue/cell availability and targeting, and therapeutic efficacy. Retinoid chemistry Retinoids are a class of compounds composed of three regions: a hydrophobic, a central polyene, and a polar (usually a carboxyl group) [29] . There are three natural retinoids: all- trans RA (ATRA), 9- cis RA (alitretinoin), and 13- cis RA (isotretinoin). To decrease the toxicity of the natural retinoids as well as to increase their stability and selectivity against a specific RAR subtype, several semi-synthetic and synthetic retinoids (including “atypical retinoids”) have been developed [29] , [30] . 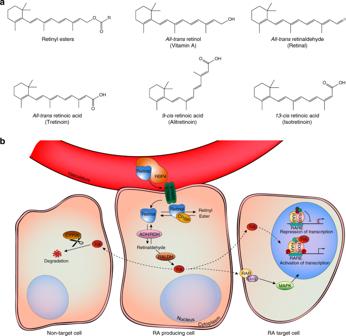Fig. 2 Retinoid chemical structures (a) and RA signaling pathway (b). Blood-circulating retinol is internalized through membrane transporter and receptorstimulated by retinoic acid 6(STRA6) and converted into all-transretinoic acid (RA), which binds to cellular retinoic acid-binding protein type 2 for signaling in the nucleus. RA triggers gene transcription by binding to RA receptors (RAR) and to the retinoid X receptor (RXR). In the presence of the ligand, RAR and RXR heterodimerize on retinoic acid-response element (RARE) sequences located in promoter regions inducing the transcription of target genes. Of note, RXR may also homodimerize and trigger gene transcription (not depicted in the illustration). RA signaling may also occur via activation of receptors associated with lipid rafts located on the cell surface, which trigger transcriptional activation of target genes by histone and receptor phosphorylation in the cell nucleus. ADH alcohol dehydrogenase, CRBP cellular retinol-binding protein 1, CYP26 cytochrome P450 family 26, Gαq Gq protein alpha subunit, MAPK mitogen activated protein kinases, P phosphorylation, RALDH retinaldehyde dehydrogenase, RBP4 retinol-binding protein 4, RDH retinol dehydrogenase. Some of them have been tested in clinical trials and approved for therapy (Table 2 ). At least four molecules have reached phase 4 clinical trials: bexarotene, tazarotene, adapalene, and trifarotene [29] , [30] , [31] . Bexarotene has optimal RXR binding, which effectively causes cancer cell death, particularly in cutaneous T-cell lymphoma. However, high levels of serum aminotransferase and liver injury have been reported [32] . Tazarotene and adapalene formulations have high affinity and selectivity for RARβ and RARγ, although the first one showed more toxicity than the second in dermatological applications [33] . Trifarotene is a selective RAR-γ agonist, approved in late 2019 in the USA, for the topical treatment of acne in patients as young as 9 years old [31] . Despite the progress made in the last years in the synthesis of novel retinoids to increase natural retinoid efficacy while reducing their toxicity, it is evident that natural retinoids are still under intense scrutiny as demonstrated by a considerable number of clinical trials (Table 1 ). The reasons are likely combinatorial: RA is a natural drug, blocks multiple disease signaling pathways [12] , in opposition to some synthetic retinoids that are very selective to a single receptor-mediated signaling pathway, and it has been used for many years in combinatorial therapy and thus well known by clinicians. Because it would be difficult to cover all advances made in retinoid delivery systems in a single review, the authors have chosen to cover only natural retinoids in the present paper. This focused approach is also supported by recent progresses in RA biology and the several formulations developed over the last years for the delivery of RA. Table 2 Synthetic retinoids in terminated or active (in bold) clinical trials and approved for commercialization. Full size table RA signaling RA is the main biologically active metabolite of vitamin A [28] . In humans, the only source of vitamin A is obtained through diet, as lipophilic retinol (or its more stable form, retinyl ester) or as carotenoids. The transport of these retinoids to cells occurs when blood-circulating retinol is bound to retinol-binding protein (RBP) 4 (Fig. 2 ). This complex interacts with membrane transporter and receptor stimulated by retinoic acid 6 facilitating entry into the cytoplasm, where retinol binds to Crbp1 (encoded by RBP1). A two-step process converts retinol into ATRA. RA binds to cellular retinoic acid-binding proteins (CRABP), assisting autocrine and paracrine signaling [34] . The mechanisms underlying paracrine signaling remain unclear while autocrine signaling requires CRABP2 for nuclear entry [28] , [34] . In the nucleus, RA triggers gene transcription by binding to heterodimers formed by RA receptors (RARα, RARβ, and RARγ) and retinoid X receptors (RXRα, RXRβ, and RXRγ). RAR–RXR heterodimers interact with a deoxyribonucleic acid sequence known as the retinoic acid-response element [35] , which facilitates the binding of co-activators to histone acetylase, ultimately leading to the transcription of target genes (Fig. 2 ). Recent data showed that RXRα homodimers can also regulate gene transcription [36] . Another isomer of RA, isomer 9- cis RA (alitretinoin), binds to retinoid X receptors [28] , [35] , while 13- cis RA (isotretinoin), has negligible affinity for retinoic acid receptors (RAR or RXR) or cellular RBP [37] . However, 13- cis RA may be converted into molecules that act as agonists for nuclear RAR and RXR. Importantly, RAR also regulates nonnuclear and nontranscriptional effects, namely the activation of kinase signaling pathways [38] (Fig. 2 ). Finally, RA is catabolized by monooxygenases of the cytochrome P450 superfamily [34] . Fig. 2 Retinoid chemical structures ( a ) and RA signaling pathway ( b ). Blood-circulating retinol is internalized through membrane transporter and receptor stimulated by retinoic acid 6 (STRA6) and converted into all- trans retinoic acid (RA), which binds to cellular retinoic acid-binding protein type 2 for signaling in the nucleus. RA triggers gene transcription by binding to RA receptors (RAR) and to the retinoid X receptor (RXR). In the presence of the ligand, RAR and RXR heterodimerize on retinoic acid-response element (RARE) sequences located in promoter regions inducing the transcription of target genes. Of note, RXR may also homodimerize and trigger gene transcription (not depicted in the illustration). RA signaling may also occur via activation of receptors associated with lipid rafts located on the cell surface, which trigger transcriptional activation of target genes by histone and receptor phosphorylation in the cell nucleus. ADH alcohol dehydrogenase, CRBP cellular retinol-binding protein 1, CYP26 cytochrome P450 family 26, Gαq Gq protein alpha subunit, MAPK mitogen activated protein kinases, P phosphorylation, RALDH retinaldehyde dehydrogenase, RBP4 retinol-binding protein 4, RDH retinol dehydrogenase. Full size image RA has very low solubility in aqueous solution (0.21 μM at pH 7.3) [18] and thus requires specific binding proteins (e.g., CRABPs) to be transported within cells to act at nuclear receptors. In addition, it has a short (few hours) lifetime, due to its degradation by a cytochrome P450-dependent monooxygenase system [39] . Moreover, it induces undesirable side effects (congenital malformations [40] as well as mucocutaneous dryness, headache, and hypertriglyceridemia [41] ) when administered at high concentrations. Therefore, for more than 35 years, several groups have developed different RA delivery systems to overcome these limitations. 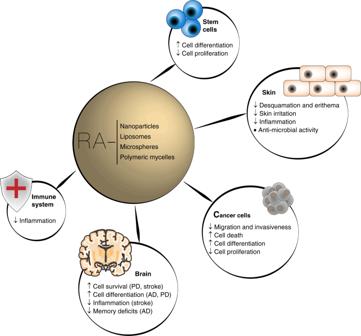Fig. 3: Main outcomes of RA-based therapies in pathological contexts. AD Alzheimer’s disease, PD Parkinson’s disease, RA retinoic acid, ↑ = increased effect, ↓ = decreased effect,●= regulatory effect. Delivery systems based in polymeric scaffolds (e.g., hydrogels, nanofibers), nanoparticles (liposomes, micelles, polymeric, dendrimers), microparticles, among others, are described and summarized in Table 3 . Table 3 Examples of formulations for the controlled release of RA in the context of cancer, brain diseases, skin diseases, immune diseases, stem cell differentiation, among other applications. Full size table Type and strategies for the delivery of RA Several strategies have been used to prepare RA delivery systems: namely, by complexation of RA with proteins (e.g., transthyretin) [42] or cationic polymers (e.g., poly(ethyleneimine) (PEI)) [43] , [44] , by physical encapsulation in polymeric [25] , [44] or inorganic [45] nanoparticles, microparticles [46] , micelles [47] , [48] , liposomes [49] , or films [43] , by covalent attachment of RA to a carrier [50] , or by immobilization of RA on surfaces of nanoparticles [45] , among others. Despite several reports on RA delivery systems based on polymeric scaffolds or electrospun fibrous meshes, the most common strategy has been based on liposomal or polymeric nanoparticles formed by polyesters, polyimines, polysaccharides, and proteins (Table 3 ). A significant number of formulations have allowed the RA encapsulation in the core of the nanoparticles. This RA encapsulation was either obtained by (1) physical or (2) chemical interaction with the components of the nanoparticle or (3) by physical entrapment. Regarding physical interaction, RA is complexed with positively charged polymers such as chitosan, or PEI [43] , [51] . The carboxylic acid of RA interacts electrostatically with the amine group located in the polymer, forming a complex that can be stabilized by addition of a polyanion and divalent ions [43] , [44] . Concerning chemical interaction, RA is typically conjugated chemically to one of the components of the nanoparticle by biodegradable ester [50] , [52] , amide [26] , [53] , [54] , [55] , or disulfide [56] linkages. These bonds are susceptible to degradation during specific pH conditions, in the presence of proteases, or reducing agents that lead to RA release. Concerning physical entrapment, RA is captured during nanoparticle formation [57] , [58] or in the pores of the nanoparticles [59] . In a relatively low number of formulations, RA was immobilized not in the core but on the surface of the nanoparticle [22] ; however, the concentration of RA immobilized on the surface is lower than in the core. Formulations with high (above 100 μg/mg of formulation) [51] , [56] , [60] , medium (between 100 and 25 μg/mg of formulation) [44] , [45] , and low (below 25 μg/mg of formulation) [7] , [58] loading have been described. The release profile of RA depends on several parameters of the formulation, including the size, composition, initial concentration of loaded RA, and its degradation profile. The sustained release of RA for more than 1 month can be accomplished by encapsulating it into biodegradable microspheres and tuning the release rate by adjusting polymer composition in the formulation [61] , by the encapsulation in polyion complex micelles [62] and adjusting polymer composition or drug content, or by the encapsulation in liposomes [49] . In general, formulations with high RA loading show a slower release profile of the drug [51] . Because of the hydrophobicity of RA, the occurrence of a burst release in most formulations is negligible [44] , [47] , [51] , [63] . Recent developments to improve the delivery of RA have led to the design of formulations that can be controlled remotely (temporally and spatially) by an external stimulus such as light, ultrasound, or magnetic forces [64] . These stimuli-responsive biomaterials are suitable for controlling the kinetic of RA delivery. In that sense, light-activatable nanoparticles containing RA that disassemble in minutes after activation by a blue laser at 405 nm have been prepared [25] , [26] , [60] . Importantly, these formulations presented higher activity than formulations in which RA was released by passive diffusion (not light triggered) because they rapidly saturated nuclear receptors. Ability of RA formulations to cross biological barriers The cellular uptake of some RA-containing nanoparticles has been demonstrated to take <12 h [44] by clathrin-mediated endocytosis and macropinocytosis [25] . Formulations that escaped the endolysosomal compartment accumulated in the cytoplasm in less than 24 h [25] , [45] . RA released in the cell cytoplasm may bind to transport proteins such as cellular retinoid-binding protein II (CRABP-II) and/or fatty acid-binding protein 5, followed by its transportation to the cell nucleus [65] . The intracellular concentration of formulations containing RA was dependent on the initial formulation loading, type of formulation, and type of cell [25] , [45] . Uptake between 25 and 80 pg of nanoparticles containing RA per cell has been described [25] . The capacity of RA-containing formulations to cross biological barriers such as the blood-brain barrier (BBB) (relevance for the treatment of brain cancer and neurodegenerative disorders) is a topic largely unexplored. In most cases, the formulations have been administered by stereotaxic and not intravenous injection [66] . Experimental data in humans indicate that ATRA administered orally is not able to accumulate in the cerebrospinal fluid [67] . Clinical trials such as NCT00528437 (Table 1 ) and others are now investigating the pharmacokinetics of 13- cis RA and its accumulation in the cerebrospinal fluid. Preclinical and clinical uses of RA formulations Formulations containing RA have been used both in preclinical and clinical trials (Fig. 3 ). Most preclinical tests were performed in mice in the context of regenerative medicine [45] , [60] , [66] , [68] and cancer [22] , [25] , [56] . In vitro tests showed that ATRA-containing liposomes [69] or ATRA-containing polymeric nanoparticles [25] , [44] were 100–1000 times more active than soluble ATRA in cultured tumor cells [25] , [69] or neural stem cells (NSC) [44] . In vivo tests showed that rats [49] or human patients [70] treated with ATRA-containing liposomes by intravenous administration had no decrease in plasma ATRA levels while animals/humans treated with oral formulation of ATRA (nonliposomal) had a significant decrease in plasma ATRA levels [41] , [49] . The results indicate that the hepatic metabolism of ATRA encapsulated in liposomes was inferior to the one observed in ATRA administered orally. Both formulations were safe in human trials. The clinical application of RA-containing formulations can be divided into two groups: (1) topical and (2) oral administration. 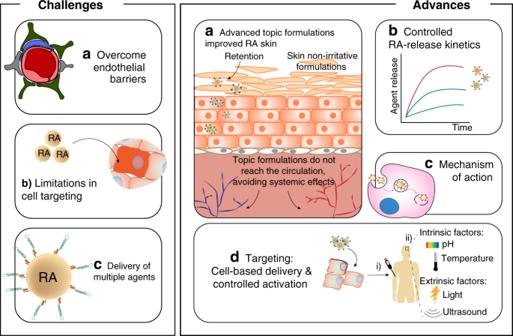Fig. 4: Challenges and advances in topical and systemic administration of RA-containing formulations. Challenges include:acrossing endothelial barriers for extravasation of RA-containing formulations into a specific body region;btargeting of RA-containing formulations to specific cells;cdevelopment of formulations that combine RA with other pharmacological agents, able to release each agent with a specific release kinetics. Advances include:adevelopment of formulations with less toxicity;brelease of RA with variable release kinetics to achieve variable biological actions;caction mechanism of RA during development and disease;duse of cells to transport RA-containing formulations to specific regions in the body followed by the triggering of the formulations by intrinsic (e.g., temperature, pH) or extrinsic (e.g., ultrasound, light) stimuli. RA retinoic acid. For topical administration, seven RA-containing formulations have reached the market for the treatment of skin-related diseases (Table 4 ). Here, current progresses are concentrated in reducing the toxicity of RA (e.g., by the use of synthetic retinoids [31] ), and exploring the combination of RA with other drugs (Table 4 ). For oral administration, four formulations containing RA have reached the market, particularly for the treatment of skin diseases (three of them) and cancer (only one) (Table 4 ). Others were tested in clinical trials but did not reach the market. For example, a liposomal-based formulation of RA (monotherapy) was successfully tested in patients with facial acne [71] and refractory hematological malignancies in a phase II clinical trial [70] . In the last application, the remission rate (67% clinical remission) was lower than that obtained using a combinatorial therapy (77% clinical remission), which included oral administration of ATRA plus idarubicin and thus the liposomal formulation was not further evaluated. Unfortunately, the liposomal formulation of RA was not tested in combination with other drugs, as it is now being investigated with nonliposomal RA formulations (Table 1 ), and this deserves further investigation in the near future. Fig. 3: Main outcomes of RA-based therapies in pathological contexts. AD Alzheimer’s disease, PD Parkinson’s disease, RA retinoic acid, ↑ = increased effect, ↓ = decreased effect, ● = regulatory effect. Full size image Table 4 Marketed RA formulations. Full size table Embryonic stem cells One of the initial applications of RA for regenerative medicine was as a differentiation agent during embryogenesis. The spatiotemporal release of RA by polymeric microparticles incorporated within embryonic bodies, derived from human embryonic stem cells, was reported to induce cell differentiation and tissue formation resembling the phenotype and structure of early human embryos [7] . Initial studies have used RA as a potent regulator of neural differentiation [72] . RA downregulates expressions of geminin and zinc finger protein Zic2, SoxB1 (Sox-1, Sox-2, Sox-3), and Notch-1, which maintain neural progenitor cell proliferation. By halting proliferation, RA shifts signaling toward differentiation. Several platforms have been used for RA delivery alone or in combination with other agents. For example, RA-containing electrospun fibrous meshes and scaffolds reportedly have an improved effect on stem cell dynamics. Electrospun poly(ε-caprolactone) fibers were loaded with ATRA, which led to extremely high local concentrations of this agent and the differentiation of murine embryonic cells, within the multilayered scaffolds [73] . Besides the neurogenic potential of RA, recent studies have highlighted the critical role of RA in the derivation of embryonic hematopoietic cells [9] , lymphoid organs [13] , and Langerhans cells that reside specifically in the epidermis [16] . Particularly, ex vivo activation of RA signaling in hemogenic endothelium, a small subpopulation of endothelial cells that can differentiate into hematopoietic cells, increased its transition into a pool of hematopoietic stem cells. Conversely, RA pathway shutdown terminated this process [9] . In addition, fetal type 3 innate lymphoid cells (ILC) are modulated by RA signaling in utero and therefore depend on appropriate maternal dietary intake of retinoids throughout pregnancy. This period also determines the ability of ILC progenitors to differentiate into mature lymphoid tissue-inducing cells [13] . It is possible that some of the RA delivery systems developed so far may be used for embryonic immune and hematopoietic stem cell development studies. Adult stem cells RA is also an important regulator of adult stem cells. For example, ATRA antagonizes stress-induced activation of dormant hematopoietic stem cells by restricting protein translation and oxidative stress [8] . When mice were fed a vitamin A-free diet to deplete the RA reservoir, animals suffered, among other effects, functional impairment of hematopoietic stem cells and their numbers were unable to recover even after injection with an immunostimulant [8] . In addition, RA-based formulations have been used as inflammatory modulators of stem cells. For example, human mesenchymal stem cells exposed to ATRA-loaded solid lipid nanoparticles significantly reduced IL-6 and IL-8 expression [74] . ATRA-containing nanoparticles have been also developed to deliver RA into NSC niches [44] . The nanoparticles had a higher effect on neuronal differentiation than solubilized RA both in vitro and in vivo [44] , [66] . The effect was mediated by an increase in transcription of the pro-neurogenic genes Ngn1 and Mash1 [44] , [66] . The formulation was then modified to remotely disassemble and release RA with spatial and temporal resolution, triggered by exposure to blue light [60] . A single short pulse of light prompted β-catenin-dependent neuronal differentiation and RARα upregulation. The combined action of blue light and RA enhanced endogenous neurogenesis. RA mode of action Several RA drugs are clinically available for dermatological treatments, including ATRA and 9- cis -RA, among others [75] . For example, 9- cis -RA encapsulated in a gel is an FDA-approved topical agent for cutaneous Kaposi’s sarcoma [75] . ATRA has also been tested in clinical trials for the treatment of the same disease [76] . This sarcoma is associated with human immunodeficiency virus infection and is characterized by a vascular endothelioma (i.e., tumor of the endothelial cells). ATRA is used clinically for treating photoaging, acne, and psoriasis. Indeed, ATRA was approved for acne vulgaris treatment in 1971 [2] , and since then, other drugs (called retinoids because they bind to RAR and/or RXR receptors) have been developed. In these clinical applications, the biological effect of ATRA includes: (1) modulation of proliferation and differentiation of skin cells; (2) anti-inflammatory activity [75] . The existence of several types of receptors and their combinations as heterodimers, as well as the ability of ATRA to modulate the activity of multiple kinase signaling pathways independently of the nuclear activation of RAR and RXR receptors, may explain the diversity of ATRA biological actions [35] . ATRA also induces skin angiogenesis and collagen deposition, increases the mitotic activity of inter- and follicular epithelium, and reduces melanin production [75] . Type of RA-containing formulations Conventional formulations containing ATRA require multiple applications to maintain the therapeutic effect. Therefore, several formulations have been developed to improve the long-term effect of ATRA, to reduce side effects like desquamation and erythema, skin irritation, and to increase the stability of RA to light [19] (Fig. 4 ). In this sense, formulations including phospholipid-based particles (e.g., solid lipid nanoparticles and nanostructured lipidic carriers) [2] , [77] , polymeric nanoparticles [2] , [27] , [77] , [78] , or polymers conjugated with RA [52] have been developed to overcome these issues. The carriers presented a particle size between 100 and 400 nm, a range of zeta potential from neutral (liposomes) to negative (polymeric nanoparticles, ethosomes, solid lipid nanoparticles, and nanostructured lipidic carriers), high entrapment efficiency (above 65%), high photostability (between two- and threefold higher than commercial tretinoin dissolved in ethanol), moderate to high skin permeation, high skin tolerance, and moderate to high antipsoriatic activity. Some of these formulations are easier to scale-up (e.g., solid lipid nanoparticles) than others [77] , [79] . In addition, some formulations (e.g., ATRA-containing liposomes) improve the local effect of RA in the skin and decrease systemic adsorption [78] . Moreover, ATRA-containing formulations increased significantly the chemical stability of ATRA during normal storage conditions (e.g., stability for 1 year at 25 °C) and after exposure to UV irradiation (twofold lower photodegradation) [77] , [80] . The protective effect of these formulations was linked to their ability to reflect and scatter UV radiation [80] . Interaction of ATRA with a lipophilic amine (stearylamine) decreases ATRA crystallinity, leading to a formulation with less skin irritating properties [77] . Fig. 4: Challenges and advances in topical and systemic administration of RA-containing formulations. Challenges include: a crossing endothelial barriers for extravasation of RA-containing formulations into a specific body region; b targeting of RA-containing formulations to specific cells; c development of formulations that combine RA with other pharmacological agents, able to release each agent with a specific release kinetics. Advances include: a development of formulations with less toxicity; b release of RA with variable release kinetics to achieve variable biological actions; c action mechanism of RA during development and disease; d use of cells to transport RA-containing formulations to specific regions in the body followed by the triggering of the formulations by intrinsic (e.g., temperature, pH) or extrinsic (e.g., ultrasound, light) stimuli. RA retinoic acid. Full size image Preclinical and clinical applications RA-containing formulations are under clinical evaluation for the treatment of acnes vulgaris , hand eczema and photoaging (Tables 1 and 3 ). An ATRA-loaded liposomal formulation has been tested in a pilot trial [71] . Patients with facial acne treated with the liposomal formulation showed higher lesion improvements than with conventional formulations. The higher efficacy of the ATRA-loaded liposomal formulation was attributed to enhanced penetration of RA across the stratum corneum . A commercial tretinoin gel microsphere formulation consisting of microspheres with 10–20 μm in size [75] has reached the market. A common issue in designing controlled RA release systems for skin applications is the limited efficacy in terms of cell targeting (Fig. 4 ). Formulations such as micro- and nanoparticles might have the capacity to target particular cells by specificities in their physicochemical properties or by incorporating in their surface peptides, proteins, or aptamers that recognize specific cell receptors. Due to their size, these formulations might accumulate preferentially in some regions of the skin, such as the follicular adduct and thus act in those biological environments. Indeed, follicular targeting is important for the treatment of acne because it increases the therapeutic effect of retinoids, while reducing their potential side effects. Polymeric micelles of diblock methoxy-poly(ethylene glycol)-poly(hexyl-substituted lactic acid) copolymer favor follicular aduct-targeted delivery of ATRA [81] . Several formulations containing RA have been used to treat Alzheimer’s disease (AD), Parkinson’s disease (PD), and stroke (Table 1 ). Current challenges in the use of RA formulations for brain diseases are ascribed to low accumulation in the brain after intravenous administration (Fig. 4 ). Although the formulations having affinity ligands in their surface have increased retention in the brain, only a minor fraction of the injected formulation reaches the brain and crosses the BBB. Cell-mediated delivery (e.g., T cells, monocytes) may be used to overcome this issue: cells can act as transporters of formulations that will be activated by local (e.g., pH) or remote triggers (e.g., light, ultrasound, magnetism) [25] , [82] once they reach the target site. Alzheimer’s disease AD is a neurodegenerative disease caused by the accumulation of amyloid-beta peptides, hyperphosphorylated tau filaments, and brain vascular changes leading to cerebral amyloid angiopathy [83] . In experimental models of AD, RA: (1) inhibited oxidative damage and mitochondrial dysfunction; (2) increased ApoE expression and suppressed inflammation; and (3) improved learning and memory [84] , [85] . Nanoparticles have been developed to efficiently deliver ATRA and small interfering RNA to promote NSC differentiation in AD [45] . In this study, the transplantation of nanoparticle-treated NSCs in AD mice improved cognition and memory. Parkinson’s disease PD is characterized by selective degeneration of dopaminergic neurons in the substantia nigra and by the accumulation of α-synuclein and Lewy bodies (protein inclusions in neurons) [68] . In experimental models of PD, RA protected against neurodegeneration of midbrain dopaminergic neurons in the substantia nigra [86] , [87] . Stereotaxic injection of ATRA-containing nanoparticles in the striatum protected nigral dopaminergic neurons in an in vivo PD model [68] . Accordingly, RA-containing nanoparticles increased expression of Nurr1 and Pitx3, key regulators of dopaminergic neuronal development and maintenance [68] , [88] . Stroke In the case of stroke, changes in the vasculature, or BBB permeability or function, may cause or enable the progression of CNS diseases [89] . RA/RAR signaling is critical for BBB differentiation and integrity [90] . Recent studies have shown protective effects of ATRA-containing nanoparticles in stroke. The formulation enhanced endothelial cell proliferation and tubule network formation and protected against ischemia-induced death in endothelial cell lines and endothelial progenitor cells isolated from ischemic stroke patients [24] . Moreover, when intravenously injected, RA formulations restored neuronal and vascular functions in a prenatal model of brain ischemia [91] . Blood cancers RA mode of action : one of the first applications of RA delivery systems was for the treatment of blood cancers. The antitumor activity of ATRA was demonstrated in 1980 in acute promyelocytic leukemia (a subtype of AML accounting for 5% of AML cases) [3] . Since then, many clinical trials have evaluated the antitumoral efficacy of the drug alone or in combination with arsenic trioxide or idarubicin [92] . RA promoted terminal differentiation of leukemic cells while reducing their proliferation. The antitumoral activity of RA (enhanced by cooperation with arsenic trioxide) [11] was due to inhibition and degradation of prolyl isomerase Pin1, which has a critical role in coordinating multiple phosphorylation events during oncogenesis [12] . Therefore, RA has the unique property of blocking multiple cancer-driving pathways simultaneously. Unfortunately, the therapeutic efficiency of ATRA-based therapies remains to be demonstrated in patients with AML without acute promyelocytic leukemia. Type of RA-containing formulations : physicochemical properties as well as release properties of RA-containing formulations for the treatment of blood cancers are summarized in Table 3 . With the exception of some formulations for parenteral administration [63] or for intracellular delivery in ex vivo conditions [25] , [26] , most RA-containing formulations have been developed for intravenous delivery. These formulations were based in liposomes [49] , [70] , [93] , microspheres [61] , polymeric micelles [63] , and nanoparticles [50] , [94] . In most cases, ATRA was encapsulated in the formulation [49] , [70] , or chemically conjugated to the carrier [50] . This effort was motivated by the fact that some of the patients treated with ATRA relapsed during the 4–6 weeks treatment of daily oral administration. Follow-up studies indicated that resistance was due to the decrease of ATRA concentration in the plasma, and thus the inability of the drug to differentiate leukemic cells [41] . The decrease was attributed to an induction of ATRA catabolism and increased levels of RA-binding protein [20] . Several ATRA delivery systems showed relative success in reducing the induction of ATRA catabolism and thus maintaining RA for longer periods in blood plasma. For example, microspheres of poly( l -lactide) showed a nearly constant release rate of ATRA for 5 weeks [61] . In addition, intravenous administration of RA-containing liposomes for 7 weeks in rats did not enhance RA catabolism [49] . Maintenance of RA in the plasma, via liposomal-encapsulated ATRA, reduced the number of relapses [95] . Targeted delivery of RA-containing formulations to the bone marrow has recently attracted much attention [96] . Bone marrow is the residence of hematopoietic stem cells that give rise to myeloid and lymphoid cell lineages. In leukemia patients, hematopoietic stem cells are the target of genetic mutations and thus aberrant activity. These altered cells are difficult to eliminate by conventional antitumoral agents because drugs do not reach the bone marrow at the required concentration, and because the stem cell niche (a physical and functional entity that supports the self-renewal and differentiation of stem cells) changes/adapts after chemotherapy, protecting altered cells [97] . RA is a potential treatment, combined with other drugs, for AML [98] and chronic myeloid leukemia [99] . In the last 10 years, a new therapeutic paradigm has emerged based on the targeted delivery of formulations to bone marrow [96] . Targeted delivery can be achieved by surface modification of nanoparticles with bisphosphonate to promote binding to bone [100] , by surface modification of liposomes with folate to target the folate receptor, which is highly expressed by AML cells [21] , [101] , by the conjugation of nanoparticles with the surface of hematopoietic stem cells [102] , or by surface modification of nanoparticles with antibodies (e.g., CD45.1, CD117) [103] , [104] or aptamers (E-selectin thioaptamer) [105] . Recently, we have developed a new platform to target bone marrow, based on light-activatable nanoparticle formulations containing ATRA [25] , [26] . The formulation was highly internalized by leukemia-initiating cells and accumulated in the cell cytoplasm. Once leukemia-initiating cells transfected with light-activatable nanoparticles containing RA were administered intravenously in leukemic mice they tend to home in the bone marrow, in the proximity of other leukemia cells. The irradiation of bone marrow with a blue light induced photo-disassembly of the nanoparticles within the cells and consequently their differentiation. These cells then secreted extracellular vesicles containing ATRA that interfered with cells supporting the stem cell niche. Preclinical and clinical applications : most RA-containing formulations are under clinical evaluation for the treatment of blood tumors (Table 1 ). Current challenges for translation of RA formulations to the clinic are related to two factors: (1) capacity to incorporate multiple drugs besides RA; (2) efficiently target hematopoietic cells (Fig. 4 ). In most cases, RA-based monotherapies are less efficient in interfering with tumorigenesis and cancer progression than combination therapies [29] . The efficiency of combination therapies is likely ascribed to several factors: (1) a combination of drugs may act at different sites of the antiproliferative signaling pathway and thus be more effective in the inhibition process; (2) combination therapies may decrease the probability of cancer resistance; (3) synergies between the drugs reduces the dose necessary for therapy, as well as their toxicity and treatment time. Currently, several clinical trials are investigating the combination of ATRA with arsenic trioxide, with arsenic trioxide and gemtuzumab ozogamicin (a monoclonal antibody against CD33 conjugated with ozogamicin, a cytotoxic agent), with epigenetic regulators such as tranylcypromine, with decitabine, cytarabine and granulocyte-stimulating factor, among others, in the context of AML (Table 1 ). Unfortunately, most RA formulations tested so far for blood cancers have not explored the simultaneous controlled release of RA and other agents. Thus, further investigation is needed to address this issue. It should be noted that a liposomal formulation having two agents (non-RA drugs) has been approved recently for AML [106] . Another important challenge in clinical translation of RA formulations is targeting. Preclinical tests have addressed different leukemia cell targets that have not yet been explored in clinical trials. The recent re-approval of gemtuzumab ozogamicin [106] may inspire new approaches for RA formulation targeting. RA delivery systems for the treatment of solid tumors RA mode of action : one of the first applications of RA formulations for the treatment of solid tumors was in mild/moderate intraepithelial cervical neoplasia [4] , [5] . ATRA was released by a collagen sponge with a cervical cap at the tumor site by insertion in the cervix. A dose of ∼ 0.4% of RA was selected for a phase II trial. Fifty percent of the patients showed a total regression of the disease [4] , [5] . Systemic and cervical side effects were mild and vaginal side effects were moderate and tolerable. Unfortunately, the formulation did not reach the market, likely because it was not sufficient to reverse or suppress more advanced dysplasia with acceptable local side effects in phase III clinical trial [107] . The antitumoral activity of RA is linked to its differentiation and cell growth arrest properties [108] . RA has been tested in several clinical trials and the results showed that RA alone did not present significant antitumoral activity against breast cancer [109] ; however, when RA was combined with tamoxifen or paclitaxel it showed moderate antitumoral activity [110] , [111] . Type of RA-containing formulations : in the last years, significant effort has been made by the scientific community to develop formulations able to release RA and other antineoplastic drugs. For example, nanoparticles containing both ATRA and paclitaxel (to inhibit cell division because the cell cannot disrupt the polymerized tubulin for cell division) had superior efficacy than formulations containing only paclitaxel [53] . In addition, pH-sensitive nanoparticles have been designed to release all- trans retinal and doxorubicin in weakly acidic tumors (pH 6.5) or acidic intracellular environments such as endosomes/lysosomes (pH 4.5–5.5) [112] . All- trans retinal was chemically conjugated to the nanoparticle polymer by hydrazone bonds that were labile under acidic conditions. Compared to free drugs, the nanoparticle formulation increased the accumulation of the all- trans -retinal and doxorubicin at the tumor site and induced higher levels of cell senescence and antitumoral activity. Progress has also been made in targeting cancer-initiating cells, which are resistant to chemotherapy and associated with tumor recurrence. ATRA liposomes and nanoparticles encapsulating simultaneously ATRA and doxorubicin have been used successfully to arrest the proliferation of breast cancer-initiating cells and to differentiate them [113] , [114] . In a combinatorial approach, RA differentiated cancer-initiating cells, whereas antineoplastic agents, such as doxorubicin, killed noncancer-initiating cells. Preclinical and clinical applications : the results of several clinical trials indicate that 13- cis RA, alone or in combination, seems to be effective at different levels against malignant gliomas [115] , and cancer occurring in the central and peripheral nervous system [116] . Moreover, ATRA inhibits proliferation of glioblastoma cells in vitro and in vivo, while promoting their differentiation [117] , [118] . At high concentrations, ATRA may induce cell apoptosis [119] . RA-coated solid lipid nanoparticles showed higher in vitro toxicity relatively to glioblastoma cells than the parent drug [120] . In addition, polymeric micelles composed by methoxy-grafted chitosan and encapsulating ATRA were more effective at inhibiting glioblastoma cell line migration in vitro than the free agent [62] . The immune system plays an important role in modulating tumor progression; however, limited infiltration of immune cells in the tumor site, as well as the existence of immunosuppressive agents, hamper their biological role. Therefore, a combination of chemotherapy with immunotherapy might be a better strategy to fight tumor biology. Indeed, immunotherapy may increase the sensitivity of cancer cells to chemotherapy and thus reduce its side effects [121] . Recently, a chemo-immunotherapy approach for melanoma was developed based on biodegradable hollow mesoporous nanoparticles containing three drugs: doxorubicin, ATRA, and interleukin (IL)-2 [23] . IL-2 is a T-cell growth factor and can thus facilitate proliferation and activation of T cells. Animals treated with formulations containing the three agents were the ones with the most effective tumor growth inhibition and decreased metastasis. ATRA was effective in differentiating myeloid-derived suppressor cells, and in synergy with doxorubicin, contributed to increase the number of dendritic cells at the tumor site; IL-2 facilitated the proliferation of CD8 + T cells at the tumor site to promote effective tumor killing. RA mode of action Inflammation is essential for the regulation of tissue homeostasis and barrier integrity (e.g., BBB, mucosal barrier). However, when dysregulated, it contributes to the pathophysiology of many diseases. In fact, retinoids have been described as potent anti-inflammatory and therefore protective in pathologies such as chronic obstructive pulmonary disease [74] , rheumatoid arthritis [122] , psoriasis [123] , and inflammatory bowel disease [124] . At a cellular level, RA inhibited IL-6-driven induction of proinflammatory Th 17 cells and promoted the differentiation of T reg cells, which are important to suppress excessive immune responses [125] . The role of RA in the gastrointestinal tract is particularly relevant since it is produced and metabolized in the intestine, where it regulates the differentiation and function of diverse immune cells and supports mucosal barrier immunity [126] . Indeed, ATRA regulates the activity of CD161 + -T reg cells that support wound repair in intestinal mucosa [14] . These C-type lectin CD161 regulatory T cells were found to induce cytokines that promoted epithelial barrier healing in the gut. Accordingly, several studies have focused on the impact of vitamin A intake (i.e., RA obtained from the diet), both during development and in the adult. Accordingly, the levels of retinoids obtained from the maternal diet increase the size of secondary lymphoid organs and the efficacy of adult immune responses [13] , while the depletion of vitamin A, in the adult, led to a decrease of Th1, Th17, and ILC3 responses (a synonym of lowered immunity to bacterial infection), an effect which is counteracted through time [127] . Type of RA-containing formulations Several RA formulations have been developed to target immune cells and induce an immunomodulatory response, such as solid lipid nanoparticles [74] , polymeric nanoparticles [58] , nanostructured lipid carriers [124] , among others. RA formulations with an average diameter of 130–250 nm [58] , [74] and an entrapment efficiency of ATRA between 2.3 and 310 μg [124] per mg of nanoparticle have been developed. Macrophage phagocytosis was influenced largely by the physicochemical properties of nanoparticles. For example, uptake is higher in nanoparticles with high negative or positive surface charges [128] . In general, RA formulations showed sustained intracellular RA delivery for a few days [58] , [74] . RA formulations are taken up by macrophages and induce anti-inflammatory responses by suppressing NF-kB signaling and increasing bone morphogenetic protein 2 signaling (pivotal for bone and cartilage development), as well as by enhancing the production of anti-inflammatory cytokines (e.g., IL-10) [58] , [124] . In addition, RA formulations have the capacity to enhance the differentiation of naïve T cells to regulatory T cells [124] . The advantages of RA-containing nanoparticles versus free RA were demonstrated by inhibiting expression of IL-6 and IL-8 in alveolar epithelial cells [74] , but were not demonstrated in the induction of immune cell differentiation. Preclinical and clinical applications Clinical trials using free RA in the context of immune thrombocytopenia (severe bleeding disorder) and sclerosing cholangitis (inflammation and scarring of the bile ducts) are active and will evaluate the role of RA as immunotherapy (Table 1 ). Current challenges for using RA formulations for immune diseases are related to the in vivo demonstration of RA effects. This requires the use of formulations able to target-specific cells, particularly immune cells, and their surface receptors (Fig. 4 ). There are classes of molecules, including antibodies, carbohydrates, peptides, aptamers that can be attached to RA formulations to target more specific immune cell populations. The advantages of RA formulations compared to free RA have been demonstrated in various biomedical applications. These are related to: (1) increased bioavailability; (2) decreased toxicity and skin irritation; (3) increased in vivo half-life; (4) increased RA photostability; (5) increased cell targeting and capacity to cross biological barriers. The advantages of RA formulations have been demonstrated in preclinical (in all applications described in this review) and clinical trials (cancer and skin applications) [71] , [129] . In the case of cancer, recent studies indicate that the antitumoral activity of RA might be greatly enhanced with formulations that extend the in vivo half-life of RA [12] . RA formulations have some limitations that preclude a more significant translation to the clinic. For example, ATRA, 9- cis -RA, and 13- cis -RA, which belong to the first generation of retinoids, are being gradually replaced in some applications by third-generation retinoids [130] . Although many of these formulations have been tested in preclinical models, the clinical translation is still relatively low. For example, although nanoparticles delivered systemically have been extensively explored in animal tests, clinical translation remains compromised because of delivery (e.g., limited efficacy in terms of cell targeting, limited capacity to cross biological barriers), technical (e.g., scale-up), and regulatory aspects (e.g., study design and approval challenges). Use of antibodies, peptides, aptamers immobilized in the surface of nanoparticles to target-specific cellular receptors may accelerate clinical translation of RA formulations. Indeed, several targeted nanoparticle formulations are now being tested in clinical trials for cancer treatment, decorated in their surface with antibodies against transferrin receptor, epidermal growth factor receptor, and ephrin type A receptor 2 [131] . In addition, the recent FDA approval of gemtuzumab ozogamicin (an antibody–drug conjugate in which the anti-CD33 antibody is linked to a cytotoxic agent) [106] or daratumumab (anti-CD38 antibody) [132] might accelerate clinical testing and the approval of other formulations conjugated with antibodies. Another issue that deserves further attention in the near future is the scale-up of the RA formulations since nanoparticles/microparticles used in most preclinical studies have been prepared in small batches. Scale-up of these formulations is challenging, as they must comply with regulatory guidelines, in terms of narrow size distribution, precise chemical composition, and drug loading [131] . In the last years, progress has been made in producing more controlled formulations with size and composition levels compatible with microfluidic systems [133] , which may advance clinical translation. Despite steady progress in the last 50 years, many issues remain to be addressed. For example, further preclinical and clinical studies are necessary to evaluate the mechanisms governing the biodistribution, pharmacokinetics, clearance, and toxicology of RA formulations. This requires the development of theranostic RA formulations that may be tracked in vivo by luminescence, magnetic resonance imaging, or positron emission tomography. Theranostic RA formulations are particularly relevant if they are injected intravenously. Moreover, further formulations should be developed with the capacity to release multiple drugs in combination with RA. Pathologies discussed in this review (neurologic diseases, cancer, immune diseases) are multifactorial and display complex signaling pathways and symptoms. Although some progress has been made in the last 5 years regarding formulations with the ability to release RA in combination with other agents [54] , [112] , further effort is needed to better control the half-life of each drug in vivo to match clinical dosage programs. Another area that deserves further investigation is the development of stimuli-responsive RA formulations that can undergo physical and/or chemical changes in response to endogenous biological or external triggers [64] . The concept here is that the systems retain the drug and release it only after a specific trigger, enhancing its therapeutic efficacy and minimizing systemic toxicity. These systems may be used for the targeted delivery of RA in hematopoietic [25] or neurogenic niches [60] . Development of these formulations requires the use of linkers susceptible to pH or enzymes present in the targeted cell/tissue. For example, several RA-polymer conjugates have been developed to release RA by hydrolytic cleavage of ester bonds [50] , [52] , by enzymatic cleavage of amide bonds by proteases present in the targeted tissue [28] , [65] , [66] , [67] or by reducing environments [56] such as the cell cytoplasm. In addition, linkers may be cleaved by an external trigger, such as light with the consequent release of RA [25] , [26] . RA is an evolutionarily ancient and conserved molecule with overlapping and pleiotropic effects. Given the diverse pharmacological activities of RA, there is ample potential for developing therapeutic applications. Thus, the fine-tuning of RA-properties and targeted formulation-based delivery is very attractive for customized and more efficient therapies. It is expected that the knowledge gathered in the development of retinoid formulations inspires others to generate delivery systems based on different drugs thus expanding the field of regenerative and therapeutic medicine.